The EutherianArmcxgenes regulate mitochondrial trafficking in neurons and interact with Miro and Trak2 Brain function requires neuronal activity-dependent energy consumption. Neuronal energy supply is controlled by molecular mechanisms that regulate mitochondrial dynamics, including Kinesin motors and Mitofusins, Miro1-2 and Trak2 proteins. Here we show a new protein family that localizes to the mitochondria and controls mitochondrial dynamics. This family of proteins is encoded by an array of armadillo (Arm) repeat-containing genes located on the X chromosome. The Armcx cluster is unique to Eutherian mammals and evolved from a single ancestor gene ( Armc10 ). We show that these genes are highly expressed in the developing and adult nervous system. Furthermore, we demonstrate that Armcx3 expression levels regulate mitochondrial dynamics and trafficking in neurons, and that Alex3 interacts with the Kinesin/Miro/Trak2 complex in a Ca 2+ -dependent manner. Our data provide evidence of a new Eutherian-specific family of mitochondrial proteins that controls mitochondrial dynamics and indicate that this key process is differentially regulated in the brain of higher vertebrates. Mitochondrial function is vital for neuronal viability, neurotransmission and neural integration [1] , [2] , [3] , [4] , [5] , [6] . Synaptic neurotransmission and integration events in nervous tissue take place at long distances from neuronal cell bodies (dendrites and axons). Consequently, to ensure energy production in distal compartments, neurons orchestrate exquisite mechanisms that regulate the transport and localization of mitochondria at active synaptic sites [7] , [8] , [9] , [10] , [11] . Mitochondrial trafficking in neurons is mediated by Kinesin and Dynein motors and by several GTPases and adaptor proteins, including Miro1/2, Trak2 or Mitofusins [12] , [13] , [14] , [15] , [16] . Mutations in genes encoding mitochondrial trafficking proteins often lead to neurological and neurodegenerative diseases [17] , [18] , [19] . Members of the Alex protein family (Alex1–3; for arm-containing protein lost in epithelial cancers linked to the X chromosome) were initially described as putative tumor-suppressor genes, as their expression is reduced in several epithelial-derived carcinomas, including lung, prostate, colon and pancreas cancers [20] . While Alex1 and 2 are widely expressed, Alex3 is found mainly in the nervous system. Previously, we characterized Alex3 as a gene preferentially expressed in the upper layers of the developing cerebral cortex [21] . A recent report described Alex3 as a Sox10-interacting protein that localizes in the mitochondria of OBL21 cells, and suggested a novel signalling cascade between the mitochondria and the nucleus through a Sox10/Alex3 protein complex [22] . Here, we describe the evolutionary history of the Armcx cluster and provide evidence that these genes encode a new family of proteins that regulates mitochondrial dynamics and that is specific to Eutherian mammals. Furthermore, we show that Alex3 protein levels affect the dynamics and trafficking of mitochondria in neurons through interaction with the Kinesin/Miro/Trak2 complex in a Ca 2+ -dependent manner. We conclude that the Armcx / Arm10 genes encode a new family of proteins that controls mitochondrial dynamics and transport in neurons. The Armcx cluster originated during the evolution of placentals To gain insight into the function of Armcx genes, we surveyed the mouse and human genomes for similar sequences. Interestingly, a full set of related genes map to the same region of the human (Xq22.1) and mouse (X56/57cM) X chromosomes, with the sole exception of the Armc10 / SVH gene, which maps to the seventh human and the fifth mouse chromosome [23] , [24] . This unusual organization prompted us to analyse further the evolutionary genesis of this gene family ( Fig. 1a ). Six homologues, named Armcx1–6 and a pseudogene ( Fig. 1a ), are arrayed in a single cluster in a portion of the X chromosome, which was proposed to be specific to placental mammals [23] , [24] . We then surveyed all available vertebrate genomes and noted the absence of Armcx genes in non-Eutherian mammals, namely monotremes and marsupials, and in non-mammalian vertebrates, and its consistent presence in all Eutherian mammals, including the earliest branching armadillo ( Supplementary Figs S1–S3 ). Hence, the Armcx cluster originated at the beginning or early radiation of the most advanced Eutherian mammals ( Fig. 1a ). Furthermore, the closest phylogenetic relative to Armcx genes, the Armc10 gene, is present in a single copy in all the vertebrate genomes analysed, including the descendants of the earliest branching mammals (monotremes and marsupials) and Eutheria. In addition, phylogenetic analyses positioned the Armc10 gene as the sister group to all Armcx genes ( Supplementary Fig. S1 and Supplementary Table S1 ), and in silico prediction emphasized the presence of up to six Arm-like repeats in the carboxy (C)-terminal region of all proteins constituting the uncharacterized DUF634 domain ( www.ebi.ac.uk/interpro/DisplayIproEntry?ac=IPR006911 ) ( Fig. 1b ). All the predicted Arm domains include the characteristic three α-helices rich in hydrophobic amino acids ( Supplementary Fig. S4 ). Furthermore, most Armcx proteins include signal peptides (such as an amino (N)-terminal signal peptide with a potential transmembrane domain), nuclear localization signals and putative mitochondrial targeting sequences ( Fig. 1b ), in agreement with our data indicating that Armcx genes are targeted to. Taken together, these observations suggest that these proteins have related physiological or cellular functions. Moreover, unusually, all Armcx-coding sequences are contained in a single exon, whereas the Armc10 is a typical, multi-exon-containing gene with the coding sequence split into at least eight exons. 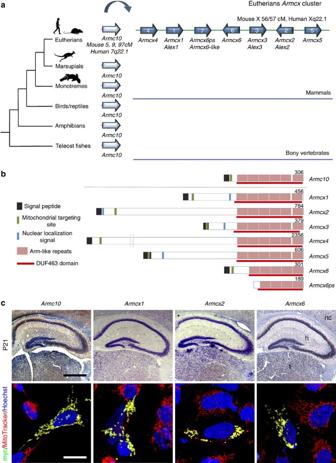Figure 1: Evolution and expression of theArmcxgene cluster. (a) Evolutionary origin of theArmcxcluster in Eutherians, through retrotransposition of the autosomalArmc10gene (curved arrow) and tandem duplication in the ancestral Eutherian X chromosome. (b) Schematic representation of the Armc10/Armcx family. They all have a highly conserved C-terminal domain (DUF463) consisting of up to six Armcx or Arm10 genes-like tandem repeats. In contrast, the N-terminal region is unrelated among members and highly variable in length and sequence, although various members share several common features, such as an N-terminal signal peptide with a potential transmembrane domain, a putative mitochondrial targeting sequence and a nuclear localization signal. (c) Expression of Armcx messenger RNAs in mouse brain and subcellular localization of Armcx proteins. The upper panels showin situhybridization demonstrating high expression ofArmc10,Armcx1,Armcx2andArmcx6genes in the hippocampus, neocortex and thalamus. The lower panels show mitochondrial targeting of Armc10, Armcx1, Armcx2 and Armcx6 proteins after transfection of Myc-tagged cDNAs in HEK293AD cells. Mitochondria were stained with the mitochondrial marker MitoTracker (red) and nuclei were stained with Hoechst (blue). Scale bars: upper panels 1 mm; and lower panels 10 μm. Figure 1: Evolution and expression of the Armcx gene cluster. ( a ) Evolutionary origin of the Armcx cluster in Eutherians, through retrotransposition of the autosomal Armc10 gene (curved arrow) and tandem duplication in the ancestral Eutherian X chromosome. ( b ) Schematic representation of the Armc10/Armcx family. They all have a highly conserved C-terminal domain (DUF463) consisting of up to six Armcx or Arm10 genes-like tandem repeats. In contrast, the N-terminal region is unrelated among members and highly variable in length and sequence, although various members share several common features, such as an N-terminal signal peptide with a potential transmembrane domain, a putative mitochondrial targeting sequence and a nuclear localization signal. ( c ) Expression of Armcx messenger RNAs in mouse brain and subcellular localization of Armcx proteins. The upper panels show in situ hybridization demonstrating high expression of Armc10 , Armcx1 , Armcx2 and Armcx6 genes in the hippocampus, neocortex and thalamus. The lower panels show mitochondrial targeting of Armc10, Armcx1, Armcx2 and Armcx6 proteins after transfection of Myc-tagged cDNAs in HEK293AD cells. Mitochondria were stained with the mitochondrial marker MitoTracker (red) and nuclei were stained with Hoechst (blue). Scale bars: upper panels 1 mm; and lower panels 10 μm. Full size image On the basis of the above data, it is likely that the entire Armcx cluster originated in early Eutherian evolution by retrotransposition of an Armc10 messenger RNA, and then by consecutive tandem duplication events in a rapidly evolving region of the Xq chromosome [23] , which also includes the Armcx-related G-protein-coupled receptor Gasp1–3 genes [24] . The precise time point for the genesis of the Armcx cluster, when key innovations of the mammalian group took place, namely the origin of a well-developed placenta, or the increase in complexity of the central nervous system and the enlargement of the neocortex [25] , suggest that this cluster has functions related to the above processes. Hence, the origin of the Armcx cluster may well have been linked to the enlargement of the neocortex, as marsupials are devoid of the Armcx cluster but have a primitive placenta. We next analysed the expression of Armcx genes during embryonic development and in the adult brain. At embryonic stages, Armc10 and Armcx3–6 genes were highly expressed in the developing neural tissues, neural crest derivatives and hind limbs, in addition to other tissues that were specific for each gene ( Supplementary Fig. S5 ). We also found that Armc10 and Armcx1–6 genes were widely expressed in the adult nervous tissue, especially in the forebrain, including the cerebral cortex, hippocampus and thalamus ( Fig. 1c ). We thus conclude that the Armcx genes encode for a Eutherian-specific set of proteins that is highly expressed in neuronal tissue. Armcx and Armc10 genes encode for mitochondrial proteins To study the subcellular localization of Armcx gene products, HEK293AD cells were transfected with complementary DNAs (cDNAs) encoding full-length Armcx proteins fused to EGFP or myc tags. In agreement with the protein domain predictions reported above, all the Alex proteins tested (Alex1, 2, 3 and 6) were targeted mainly to mitochondria, which were visualized by cellular staining with MitoTracker ( Fig. 1c ; and Supplementary Fig. S6 ). Nuclear staining was also occasionally seen in individual cells. Transfection with a cDNA encoding Armc10 yielded an identical pattern of mitochondrial staining ( Fig. 1c ). Many cells transfected with Armcx1, 2, 3 and 6 and Armc10 cDNAs showed an altered mitochondrial network, in which mitochondria were aggregated in the perinuclear region ( Fig. 2a and Supplementary Fig. S6 ). We conclude that the Armc10/Armcx cluster encodes for a new family of proteins targeted to mitochondria and possibly regulates the dynamics and distribution of these organelles. 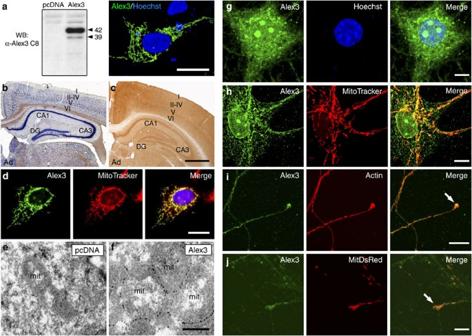Figure 2: Expression and localization of Alex3 protein. (a) Anti-Alex3 antibody specifically recognizes Alex3 protein. The antibody recognizes two specific species of about 42 and 39 KDa in HEK293AD cells transfected with Armcx3 cDNA, as shown in WB (left panel). Immunocytochemical detection of Alex3 protein in transfected cells (right panel). (b,c) Coronal sections of adult mouse forebrain showing similar patterns of expression of Armcx3 transcripts (b) and Alex3 protein (c) in the neocortex and hippocampus. (d) Confocal images showing that Alex3 (green) colocalizes with mitochondria in HEK293AD cells; cells were stained with MitoTracker. (e,f) Electron microscopy images of HEK293AD cells transfected with an empty vector (e) or with an Alex3 expression vector (f), illustrating Alex3 localization (gold particles) around mit. (g–j) Immunolocalization of Alex3 protein in cultured hippocampal neurons at 15 DIV. Endogenous Alex3 shows a heterogeneous distribution. Alex3 (green) localizes in nuclei, as shown by colabelling with the nuclear marker Hoechst (blue) (g); in the cytoplasm, Alex3 signals show a punctate pattern that corresponds to the mitochondrial compartment stained with MitoTracker (red) (h); in the cytosol, Alex3 colocalizes with Phalloidin staining (red), particularly in growth cones (arrow) (i). (j) Alex3 staining decorates mitochondria (labelled with MitDSRed) in growth cones. CA1–CA3: Cornu Ammonis1–3; DG: dentate gyrus; I–II–III–IV–V–VI: neocortical layers; mit: mitochondria. Scale bars: 1 mm (b,c); 15 μm (a,c,d); 5 μm (g,h,i,j); and 0.02 μm (e,f). Figure 2: Expression and localization of Alex3 protein. ( a ) Anti-Alex3 antibody specifically recognizes Alex3 protein. The antibody recognizes two specific species of about 42 and 39 KDa in HEK293AD cells transfected with Armcx3 cDNA, as shown in WB (left panel). Immunocytochemical detection of Alex3 protein in transfected cells (right panel). ( b , c ) Coronal sections of adult mouse forebrain showing similar patterns of expression of Armcx3 transcripts ( b ) and Alex3 protein ( c ) in the neocortex and hippocampus. ( d ) Confocal images showing that Alex3 (green) colocalizes with mitochondria in HEK293AD cells; cells were stained with MitoTracker. ( e , f ) Electron microscopy images of HEK293AD cells transfected with an empty vector ( e ) or with an Alex3 expression vector ( f ), illustrating Alex3 localization (gold particles) around mit. ( g – j ) Immunolocalization of Alex3 protein in cultured hippocampal neurons at 15 DIV. Endogenous Alex3 shows a heterogeneous distribution. Alex3 (green) localizes in nuclei, as shown by colabelling with the nuclear marker Hoechst (blue) ( g ); in the cytoplasm, Alex3 signals show a punctate pattern that corresponds to the mitochondrial compartment stained with MitoTracker (red) ( h ); in the cytosol, Alex3 colocalizes with Phalloidin staining (red), particularly in growth cones (arrow) ( i ). ( j ) Alex3 staining decorates mitochondria (labelled with MitDSRed) in growth cones. CA1–CA3: Cornu Ammonis1–3; DG: dentate gyrus; I–II–III–IV–V–VI: neocortical layers; mit: mitochondria. Scale bars: 1 mm ( b , c ); 15 μm ( a , c , d ); 5 μm ( g , h , i , j ); and 0.02 μm ( e , f ). Full size image To gain insight into the functional role of Alex proteins, we focussed on Alex3 [21] . We generated antibodies against a synthetic peptide corresponding to the Alex3 sequence. Following transfection of Alex3 in HEK293AD cells, these antibodies recognized this protein in western blots (WBs) and immunofluorescence ( Fig. 2a ). A similar band was detected in WBs of brain lysates ( Supplementary Fig. S7 ). The regional and cellular pattern of Alex3 immunostaining in brain sections was identical to that found in in situ hybridization analyses ( Fig. 2b,c ). Thus, Alex3 protein was widely expressed in most brain regions and neurons; Alex3 protein expression peaked at postnatal stages (P0–P21) and decreased slightly thereafter. In transfected HEK293AD cells, Alex3 immunostaining colocalized with mitochondria, where Alex3 signals appeared to wrap individual mitochondria ( Fig. 2d ; Supplementary Fig. S8a,b ). Immunogold electron microscopy confirmed that Alex3 protein surrounded mainly the outer mitochondrial membrane ( Fig. 2e,f ). These observations are consistent with a previous study reporting Alex3 protein in outer membrane mitochondrial fractions [22] . To identify the protein regions required for this targeting, we generated truncated Alex3–EGFP constructs. Transfection with deletions at the C-terminus produced a mitochondrial localization pattern that was indistinguishable from that observed with the full-length Alex3–green fluorescent protein (GFP) cDNA. In contrast, a deleted construct at the N-terminus (GFP–Alex3Δ1–12) abolished mitochondrial targeting and led to nuclear localization. Moreover, we found that the Arm-containing domains are not required for mitochondrial targeting ( Supplementary Fig. S8b–e ). We conclude that the N-terminal sequence of Alex3 is necessary and sufficient to target the Alex3 protein to the mitochondrial network. We next examined the distribution of Alex3 protein in cultured hippocampal neurons. These cells exhibited strong cytosolic Alex3 signals, which colocalized with the mitochondrial network in cell bodies, axons and dendrites ( Fig. 2g,h ). In addition, Alex3 signals were distributed throughout the cytosol and showed strong colocalization with the actin cytoskeleton, particularly in neurites and growth cones, where Alex3 also colocalized with mitochondria ( Fig. 2i,j ). Finally, many neurons exhibited Alex3 immunostaining in nuclei ( Fig. 2g ). We conclude that endogenous Alex3 is localized in three neuronal pools: mitochondria, nucleus and cytosol. Alex3 regulates mitochondrial network and aggregation To study whether Alex3 proteins regulate the bioenergetic mitochondrial state or Ca 2+ handling, we performed several experiments. First, we found that overexpression of Alex3 in HEK293T cells did not alter O 2 consumption or DNA copy number ( Fig. 3a,b ). These data, together with findings in neurons showing that Alex3 protein levels do not modify COX/citrate synthase ratios, DNA copy number or mitochondrial membrane potential ( Fig. 3c–e ), indicate that this protein is not involved in the regulation of bioenergetic mitochondrial parameters. To examine whether Alex3 controls mitochondrial Ca 2+ handling [26] , we transfected cells with a mitochondria-targeted aequorin/GFP fusion protein [27] , and measured mitochondrial uptake of Ca 2+ . Our data show that neither the uptake of Ca 2+ released from the endoplasmic recticulum (ER) by stimulation with ATP+carbachol nor mitochondrial Ca 2+ uptake by cells whose plasma membrane had been permeabilized by treatment with digitonin was altered by the overexpression of Alex3 ( Fig. 3f,g ). 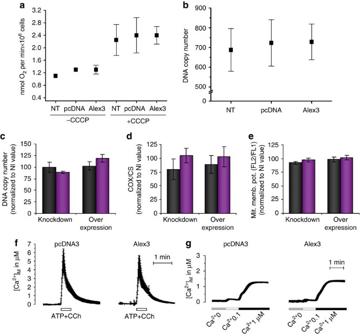Figure 3: Neither overexpression nor knockdown of Alex3 impairs the bioenergetic mitochondrial parameters or Ca2+handling. HEK293T cells (a,b) were transfected with Alex3 or pcDNA3–control, and the oxygen consumption (a) and mitochondrial DNA copy number (b) were measured. There were no differences between control (pcDNA3 or non-transfected (NT) cells) and Alex3-overexpressing cells (a,b). When the uncoupling protein CCCP was added to the medium, oxygen consumption increased but again the differences were not statistically significant. (c,e) Hippocampal neurons were infected with pWPI (control; black bars) and pWPI–Alex3 (purple bars) in overexpression experiments, and shRNAi–control (black bars) or shRNAi–Alex3 (purple bars) in knockdown experiments. After 7 days, we measured mitochondrial DNA copy number (c), COX and citrate synthase activity (d) and mitochondrial membrane potential (mit. memb. pot.) (e) (JC1 assay, ratio between red (Fl2) and green (FL1) fluorescence). The values were normalized against values from non-infected neurons (NI). No significant differences were found in any of the above parameters. The values show mean±s.e.m. from three independent experiments. (f,g) Mitochondrial Ca2+uptake in HEK293T cells transfected with mitochondria-targeted aequorin (see Methods) together with Alex3 (or pcDNA3 in the control). (f) Intact cells were stimulated by ATP+CCh (100 μM each) to trigger maximum IP3-induced Ca2+release from the ER. Because of extremely close coupling between ER and mitochondria, much of this released Ca2+is taken up by the mitochondrial Ca2+uniporter. There were no significant differences between control (pcDNA3) and Alex3 conditions. (g) The mitochondrial uptake from intracellular-like medium was directly measured in cells permeabilized with 60 μM digitonin for 1 min in Ca2+-free solution (see Methods). Then perfusion was switched first to 0.1 μM Ca2+, which is insufficient to activate the mitochondrial uniporter, and then to 1 μM Ca2+, which promotes some mitochondrial Ca2+uptake. Uptake was similar in control and Alex3-transfected cells in all experimental conditions. Data represent mean±s.e.m. from 4–5 independent experiments. Figure 3: Neither overexpression nor knockdown of Alex3 impairs the bioenergetic mitochondrial parameters or Ca 2+ handling. HEK293T cells ( a , b ) were transfected with Alex3 or pcDNA3–control, and the oxygen consumption ( a ) and mitochondrial DNA copy number ( b ) were measured. There were no differences between control (pcDNA3 or non-transfected (NT) cells) and Alex3-overexpressing cells ( a , b ). When the uncoupling protein CCCP was added to the medium, oxygen consumption increased but again the differences were not statistically significant. ( c , e ) Hippocampal neurons were infected with pWPI (control; black bars) and pWPI–Alex3 (purple bars) in overexpression experiments, and shRNAi–control (black bars) or shRNAi–Alex3 (purple bars) in knockdown experiments. After 7 days, we measured mitochondrial DNA copy number ( c ), COX and citrate synthase activity ( d ) and mitochondrial membrane potential (mit. memb. pot.) ( e ) (JC1 assay, ratio between red (Fl2) and green (FL1) fluorescence). The values were normalized against values from non-infected neurons (NI). No significant differences were found in any of the above parameters. The values show mean±s.e.m. from three independent experiments. ( f , g ) Mitochondrial Ca 2+ uptake in HEK293T cells transfected with mitochondria-targeted aequorin (see Methods) together with Alex3 (or pcDNA3 in the control). ( f ) Intact cells were stimulated by ATP+CCh (100 μM each) to trigger maximum IP3-induced Ca 2+ release from the ER. Because of extremely close coupling between ER and mitochondria, much of this released Ca 2+ is taken up by the mitochondrial Ca 2+ uniporter. There were no significant differences between control (pcDNA3) and Alex3 conditions. ( g ) The mitochondrial uptake from intracellular-like medium was directly measured in cells permeabilized with 60 μM digitonin for 1 min in Ca 2+ -free solution (see Methods). Then perfusion was switched first to 0.1 μM Ca 2+ , which is insufficient to activate the mitochondrial uniporter, and then to 1 μM Ca 2+ , which promotes some mitochondrial Ca 2+ uptake. Uptake was similar in control and Alex3-transfected cells in all experimental conditions. Data represent mean±s.e.m. from 4–5 independent experiments. Full size image During the above experiments, we noted that cells transfected with Alex3 (as well as with Alex1, 2 and 6 and Armc10) exhibited altered mitochondrial networks ( Fig. 4a,b and Supplementary Fig. S6 ). To further explore this observation, HEK293AD cells were transfected with Alex3 and the mitochondrial morphology of these cells was monitored 2 days later ( Fig. 4a ). We found that 88% of these cells presented abnormal, aggregated-like mitochondrial networks. Of these cells, 33% showed strongly aggregated phenotypes, in which virtually all the mitochondria were concentrated in large, single aggregates near the nucleus; the remaining 55% showed variable and intermediate degrees of clustered mitochondria ( Fig. 4a,c ). The severity of the mitochondrial phenotype correlated with the expression levels of Alex3 protein ( Supplementary Fig. S9 ), in a way similar to that found in Mitofusin 1-overexpressing cells [28] . We also imaged Alex3–GFP-transfected cells over 6 h. Concomitant to Alex3–GFP expression, individual mitochondria aggregated to finally form one or two large clusters ( Fig. 4d and Supplementary Movie 1 ). Furthermore, electron microscopy analysis confirmed that the overexpression of Alex3 causes the aggregation of mitochondria ( Fig. 4e,f ). 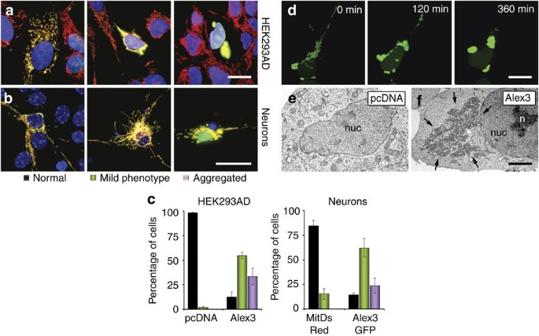Figure 4: Alex3 overexpression severely alters mitochondrial morphology and distribution leading to a perinuclear aggregation. (a,b) Overexpression of Alex3 in HEK293AD (a) or Alex3–GFP in 12 DIV hippocampal neurons (b) induces severe alterations in the morphology and distribution of the mitochondrial net when compared with the expression of a control vector (pcDNA in HEK293AD or MitDsRed in neurons). We classified these effects on a 3-point scale from no substantial changes as shown in the first column, a wide spectrum of severe alterations illustrated in the second column and to the most severe phenotype, consisting of the complete aggregation of the mitochondrial net in the perinuclear region, as presented in the third column. (c) Quantification and graphical representation (mean±s.d.) of the above mentioned subpopulations of Alex3- or ALEX3–GFP-overexpressing cells. We counted 167–345 HEK293 cells and 51–116 neurons per single experiment. Data represent two and three independent experiments, respectively. (d) Series of time-lapsed images of an Alex3–GFP-overexpressing HEK293AD cell showing mitochondrial aggregation. (e,f) Electron microscopy micrographs of HEK293AD cells overexpressing a control vector (e) or Alex3 protein (f). Images show mitochondrial aggregates and their location near the nucleus (d). n: nucleolus; nuc: nucleus. Scale bars: 15 μm (a,b,d); and 2 μm (e,f). Figure 4: Alex3 overexpression severely alters mitochondrial morphology and distribution leading to a perinuclear aggregation. ( a , b ) Overexpression of Alex3 in HEK293AD ( a ) or Alex3–GFP in 12 DIV hippocampal neurons ( b ) induces severe alterations in the morphology and distribution of the mitochondrial net when compared with the expression of a control vector (pcDNA in HEK293AD or MitDsRed in neurons). We classified these effects on a 3-point scale from no substantial changes as shown in the first column, a wide spectrum of severe alterations illustrated in the second column and to the most severe phenotype, consisting of the complete aggregation of the mitochondrial net in the perinuclear region, as presented in the third column. ( c ) Quantification and graphical representation (mean±s.d.) of the above mentioned subpopulations of Alex3- or ALEX3–GFP-overexpressing cells. We counted 167–345 HEK293 cells and 51–116 neurons per single experiment. Data represent two and three independent experiments, respectively. ( d ) Series of time-lapsed images of an Alex3–GFP-overexpressing HEK293AD cell showing mitochondrial aggregation. ( e , f ) Electron microscopy micrographs of HEK293AD cells overexpressing a control vector ( e ) or Alex3 protein ( f ). Images show mitochondrial aggregates and their location near the nucleus ( d ). n: nucleolus; nuc: nucleus. Scale bars: 15 μm ( a , b , d ); and 2 μm ( e , f ). Full size image To study whether that Alex3 overexpression also leads to mitochondrial aggregation in neurons, we transfected hippocampal cultures ( Fig. 4b,c ). Up to 85% of Alex3–GFP-transfected neurons exhibited an abnormal mitochondrial phenotype; 23% of neurons displayed mitochondria completely aggregated in perinuclear clusters, whereas the remaining 62% of neurons displayed intermediate phenotypes with mildly aggregating mitochondria. These phenotypes were not found in control neurons ( Fig. 4c ). To confirm that Alex3 causes aggregation, we studied the fine structure of mitochondrial networks in Alex3-transfected hippocampal neurons ( Supplementary Fig. S10 ). These cells displayed large aggregates of mitochondria in the cell bodies, in which individual mitochondria, surrounded by Alex3-immunoreactive end product, were clearly identifiable. Examination of the neurites also showed the presence of elongated aggregated mitochondria. Taken together, the above data suggest that the Armc10 / Armcx gene cluster (and particularly Armcx3) encodes for proteins involved in mitochondrial aggregation and dynamics. To directly test whether Alex3 regulates mitochondrial fusion, we took advantage of a photoactivable mito-PAGFP version [29] . HEK293T cells transfected with mito-PAGFP were photoactivated and video recorded over 15 min, and the rates of mitochondrial fusion were analysed (yellow channel; Fig. 5a,b ). In agreement with previous studies [29] , [30] , [31] , we observed a constant increase in mitochondrial fusion events over time ( Supplementary Movies 2 and 3 ). The rate and dynamics of these events in cells transfected with Alex3 were identical to those in control cells ( Fig. 5c ; Supplementary Fig. S11 ). Similar experiments in hippocampal neurons, either overexpressing Alex3 or a shRNA sequence, gave similar results ( Fig. 5d and Supplementary Movies 4 and 5 ). 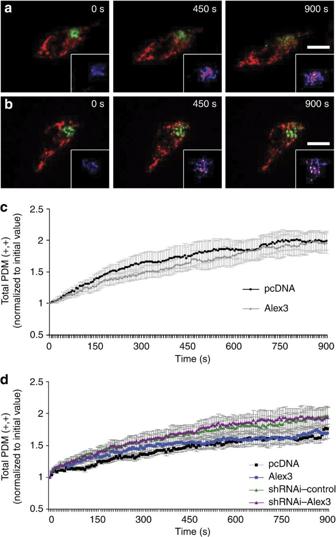Figure 5: Alex3 protein does not alter mitochondrial fusion. (a,b) HEK293T cells were transfected with MitDsRed, mito-PAGFP and pcDNA (a), or Alex3 (b). Mito-PAGFP was photoactivated, MitDsRed was photobleached att=0 s, and cells were video recorded over 15 min. Panels in (a,b) show the same cell at a range of time points; note the increase in yellow signals representing mitochondrial fusion (insets). The rates of fusion were analysed (c) using PDM (+,+) images (shown in boxed areas in (a,b)). Eleven cells, corresponding to two independent experiments, were quantified for each group. (d) Rates of mitochondrial fusion over time in hippocampal neurons overexpressing Alex3, or a shRNA, demonstrating that Alex3 levels do not alter mitochondrial fusion in neurons. At least eight cells, corresponding to two independent experiments, were quantified for each group. The values show mean±s.e.m. Scale bar: 15 μm. Figure 5: Alex3 protein does not alter mitochondrial fusion. ( a , b ) HEK293T cells were transfected with MitDsRed, mito-PAGFP and pcDNA ( a ), or Alex3 ( b ). Mito-PAGFP was photoactivated, MitDsRed was photobleached at t =0 s, and cells were video recorded over 15 min. Panels in ( a , b ) show the same cell at a range of time points; note the increase in yellow signals representing mitochondrial fusion (insets). The rates of fusion were analysed ( c ) using PDM (+,+) images (shown in boxed areas in ( a , b )). Eleven cells, corresponding to two independent experiments, were quantified for each group. ( d ) Rates of mitochondrial fusion over time in hippocampal neurons overexpressing Alex3, or a shRNA, demonstrating that Alex3 levels do not alter mitochondrial fusion in neurons. At least eight cells, corresponding to two independent experiments, were quantified for each group. The values show mean±s.e.m. Scale bar: 15 μm. Full size image As Miro1 interacts with Alex3 (see below) and has been shown to control mitochondrial aggregation [32] , [33] , we tested whether this protein mediates the mitochondrial aggregation phenotype induced by Alex3. We observed that downregulation of Miro1 protein did not alter the aggregating phenotype caused by Alex3 ( Supplementary Fig. S12 ). Taken together, our data indicate that Alex3 regulates mitochondrial aggregation, rather than mitochondrial fusion, by mechanisms independent of Miro1. Alex3 regulates mitochondrial trafficking in neurons Mitochondrial transport is essential for neuronal viability [18] , [19] , [34] , [35] . To address whether Alex3 is involved in mitochondrial transport in axons, we used live-imaging techniques. Cultured hippocampal neurons were transfected at 4 DIV with mitochondrial-targeted DsRed (MitDsRed) or Alex3–GFP. After 2 days, axons were identified and recorded over 15 min ( Fig. 6 ). Control neurons exhibited high motility rates for mitochondria, which were transported both in the anterograde and retrograde directions ( Fig. 6a,b and Supplementary Movie 6 ). As described [8] , only a fraction of individual mitochondria (about 30%, Fig. 6e ) moved over the 15-min recording periods, whereas the remaining ones remained stationary. The distance covered in single trafficking events by mitochondria was heterogeneous. While some organelles moved over relatively long distances (more than 100–150 μm), others displaced only a few μm (10–20 μm). The speed at which single mitochondria were transported was also variable (anterograde: average=0.21±0.14 μm per segment; range: 0.07/ 1.03 μm per segment; retrograde: average=0.29±0.15 μm per segment; range 0.07/0.83 μm per segment). Mitochondrial trafficking tended to be more active in the retrograde than in the anterograde direction ( Fig. 6e ). 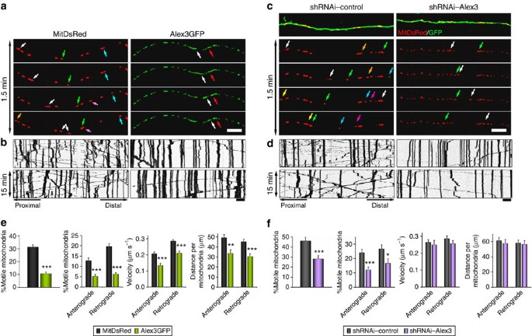Figure 6: Alex3 protein levels regulate axonal transport of mitochondria in hippocampal neurons. (a,c) Series of four representative confocal images, taken every 30 s, of live axons overexpressing the mitochondrial-tagged protein MitDsRed or Alex3–GFP fusion protein (a), or MitDsRed plus a control shRNAi or a specific Alex3 shRNAi (c). Coloured arrows identify the same mitochondria through the different acquisitions. (c) The upper panel identifies the imaged axon expressing GFP after infection. (b,d) Representative kymographs (two per condition) showing the full-time acquisition periods (that is, 15 min of movie) in overexpressing (c) and in silencing experiments (d). All kymographs are arranged with the distal axonal end to the right. (e,f) Graphical representation of the percentage of motile mitochondria, velocity and distance covered by individual mitochondria measured in kymographs for the overexpression (e) or silencing (f) experiments. Data were analysed using the Student'st-test and represent the mean±s.e.m of 22–42 axons (neurons) per experimental group, from at least eight independent experiments. ***P<0.001; **P<0.01; *P<0.05 (For individualPsee text). Scale bars: 10 μm. Figure 6: Alex3 protein levels regulate axonal transport of mitochondria in hippocampal neurons. ( a , c ) Series of four representative confocal images, taken every 30 s, of live axons overexpressing the mitochondrial-tagged protein MitDsRed or Alex3–GFP fusion protein ( a ), or MitDsRed plus a control shRNAi or a specific Alex3 shRNAi ( c ). Coloured arrows identify the same mitochondria through the different acquisitions. ( c ) The upper panel identifies the imaged axon expressing GFP after infection. ( b , d ) Representative kymographs (two per condition) showing the full-time acquisition periods (that is, 15 min of movie) in overexpressing ( c ) and in silencing experiments ( d ). All kymographs are arranged with the distal axonal end to the right. ( e , f ) Graphical representation of the percentage of motile mitochondria, velocity and distance covered by individual mitochondria measured in kymographs for the overexpression ( e ) or silencing ( f ) experiments. Data were analysed using the Student's t -test and represent the mean±s.e.m of 22–42 axons (neurons) per experimental group, from at least eight independent experiments. *** P <0.001; ** P <0.01; * P <0.05 (For individual P see text). Scale bars: 10 μm. Full size image We recorded only Alex3–GFP-tranfected neurons that displayed an apparently normal distribution of mitochondria in the cell bodies and in axons. In these cultures, Alex3–GFP protein was targeted mainly to mitochondria and virtually all the mitochondrial meshwork displayed Alex3 signals ( Fig. 6a and Supplementary Fig. S13 ). We also noted that individual mitochondria were larger in Alex3–GFP-transfected neurons than in control cells ( Fig. 6a and Supplementary Fig. S14a ). Examination of video recordings indicated that mitochondrial transport was reduced in these neurons. To confirm this observation, video recordings were represented as kymographs [36] and mitochondrial motility was analysed quantitatively ( Fig. 6b,e ). Overexpression of Alex3–GFP resulted in a dramatic reduction in the percentage of moving mitochondria, in both the anterograde and retrograde directions ( Fig. 6e and Supplementary Movie 7 ). This effect was independent of mitochondrial size ( Supplementary Fig. S15 ). Moreover, the velocity and average distance covered by individual mitochondria was impaired in neurons overexpressing Alex3–GFP ( Fig. 6e ). To confirm the involvement of Alex3 in mitochondrial dynamics and trafficking, we performed experiments to knockdown endogenous Alex3 protein. Hippocampal neurons were transfected with pLVTHM vectors expressing shRNAi-Alex3 sequences ( Supplementary Fig. S16 ), or a control scrambled sequence. Neurons expressing shRNAi for Alex3 transcripts were viable and morphologically normal, and they extended normal dendrites and axons ( Supplementary Fig. S17 ). Alex3–shRNAi-expressing neurons exhibited reduced mitochondrial motility and trafficking and smaller mitochondria than control neurons ( Fig. 6c,d , Supplementary Movies 8 , 9 , and Supplementary Fig. S14b ). This decrease was for anterograde and retrograde transport. However, neither the velocity nor the distance covered by single movements of individual mitochondria was altered by the knockdown of endogenous Alex3 ( Fig. 6f ). Taken together, these experiments show that Alex3 expression levels regulate the motility of mitochondria in axons in living neurons and modulate both the velocity and distance covered by these organelles. Alex3 interacts with Miro and Trak2 proteins Mitochondrial trafficking in neurons is mediated by Kinesin (KIF5) motors [37] , by the Kinesin adaptor Trak2 and by the Rho GTPases Miro1 and Miro2 [14] , [38] . We next studied whether Alex3 forms part of the KIF5/Miro/Trak2 trafficking complex. First, immunofluorescence analyses in transfected HEK293AD cells showed strong colocalization of Alex3 with Miro1, Miro2 and Trak2, while no apparent colocalization was detected with KIF5C ( Supplementary Fig. S18 ). Next, we performed co-immunoprecipitation assays in HEK293AD cells transfected with Alex3–GFP and either Miro1-myc or Miro2-myc cDNAs. Miro1 and Miro2 were detected by WB in lysates immunoprecipitated with anti-GFP antibodies. Conversely, pull-downs with anti-myc antibodies revealed Alex3–GFP protein. No co-immunoprecipitation was detected when cells were transfected with either Miro1/2-myc or Alex3–GFP DNA alone ( Fig. 7a ). Similar experiments showed that Alex3–GFP was co-immunoprecipitated with Trak2-myc protein ( Fig. 7c ). In contrast, we did not detect co-immunoprecipitation of Alex3–GFP with KIF5C, KIF5A or KIF5B ( Fig. 7b ). These data indicate that Alex3 interacts directly with the Miro1-2/Trak2 proteins, thereby suggesting that this protein is therefore involved in the KIF5/Miro/Trak2 trafficking complex. 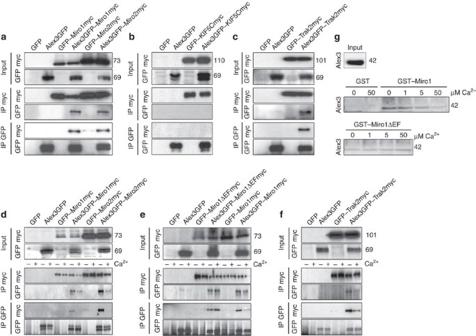Figure 7: Alex3 is a component of the protein complex responsible for mitochondrial transport. (a–f) A GFP construct was used as control. (a–c) Co-immunoprecipitation of Alex3–GFP with Miro1myc, Miro2myc, KIF5Cmyc or Trak2myc results in the specific interaction of Alex3–GFP with Miro1myc, Miro2myc (a) and Trak2myc (c) but no interaction is detected between Alex3–GFP and KIF5Cmyc (b). (d) The interaction between Alex3–GFP and Miro1myc and Miro2myc is reduced in the presence of 2 mM of calcium. (e) When the EF-hand mutant form of Miro1myc is co-expressed with Alex3–GFP, the interaction between the two components is no longer sensitive to Ca2+levels. (f) The association between Alex3–GFP and Trak2myc is also dependent on the presence of Ca2+, thereby indicating that the whole complex could be dismantled when Miro1/2 recognizes an increment in Ca2+levels. (g) Pull-down assays using purified GST–Miro1 and GST–Miro1ΔEF proteins as bait and showing interaction with Alex3 (in brain lysates) and its dependence on Ca2+concentration (top panel). The lack of the EF-hand domain in Miro-1 protein abolishes Ca2+dependence (bottom panel). Figure 7: Alex3 is a component of the protein complex responsible for mitochondrial transport. ( a – f ) A GFP construct was used as control. ( a – c ) Co-immunoprecipitation of Alex3–GFP with Miro1myc, Miro2myc, KIF5Cmyc or Trak2myc results in the specific interaction of Alex3–GFP with Miro1myc, Miro2myc ( a ) and Trak2myc ( c ) but no interaction is detected between Alex3–GFP and KIF5Cmyc ( b ). ( d ) The interaction between Alex3–GFP and Miro1myc and Miro2myc is reduced in the presence of 2 mM of calcium. ( e ) When the EF-hand mutant form of Miro1myc is co-expressed with Alex3–GFP, the interaction between the two components is no longer sensitive to Ca 2+ levels. ( f ) The association between Alex3–GFP and Trak2myc is also dependent on the presence of Ca 2+ , thereby indicating that the whole complex could be dismantled when Miro1/2 recognizes an increment in Ca 2+ levels. ( g ) Pull-down assays using purified GST–Miro1 and GST–Miro1ΔEF proteins as bait and showing interaction with Alex3 (in brain lysates) and its dependence on Ca 2+ concentration (top panel). The lack of the EF-hand domain in Miro-1 protein abolishes Ca 2+ dependence (bottom panel). Full size image To determine whether the Arm-like domains of Alex3 were required for interaction with these proteins, we generated a N-terminus Alex3(1-106) construct lacking the six Arm domains. Co-immunoprecipitation experiments in HEK293T cells showed that this mutant protein did not co-immunoprecipitate with Trak2 or Miro2 proteins ( Supplementary Fig. S19 ), thereby indicating that the Arm-containing C-terminal region is required for this interaction. The Miro/Trak2 complex interacts with Kinesin motors in a Ca 2+ -dependent manner, in which Ca 2+ binding to Miro proteins triggers the uncoupling of the complex to microtubules, thereby allowing mitochondrial arrest [10] , [11] . We thus tested whether the association of Alex3 with the trafficking complex was also Ca 2+ -dependent. The presence of 2 mM Ca 2+ markedly reduced the interaction of Alex3 with Miro1, 2 and Trak2 ( Fig. 7d,e ). Interestingly, cotransfection of Alex3–GFP with a Miro1-myc mutant cDNA lacking the EF-hand domain responsible for Ca 2+ binding blocked the regulation of Miro1/Alex3 interaction by Ca 2+ , thereby reinforcing the notion that the interaction between these two proteins is regulated by Ca 2+ levels ( Fig. 7f ). To corroborate these findings, we purified GST-Miro1 protein and performed pull-downs with extracts from brain lysates [10] . These experiments confirmed the direct interaction of Alex3/Miro1 proteins, as well as the regulation of this interaction by Ca 2+ and the dependence on the EF-hand domain in Miro1 protein for the regulation of the complex by Ca 2+ ( Fig. 7g ). Taken together, the above data demonstrate that Alex3 belongs to the KIF5/Miro1-2/Trak2 mitochondrial trafficking complex and that the Alex3/Miro1 protein interaction requires low Ca 2+ concentrations. Mitochondrial dynamics is essential for neuronal viability and neurotransmission. Moreover, neuronal mitochondrial dynamics is highly coordinated and largely controlled by Kinesins, the GTPases Mitofusins1–2 and Miro1–2, and the adaptor protein Trak2 [3] , [12] , [31] . Here we describe a family of proteins targeted to mitochondria that controls the distribution and dynamics of these organelles and that is evolutionarily specific for Eutherian mammals. The Armcx gene cluster arose by retrotransposition from a single Arm-containing gene ( Armc10 ) exclusive to and present in all vertebrates, and by subsequent short-range tandem duplications of a rapidly evolving region of the Eutherian X chromosome. Given that the expression of retrotransposed genes depends largely on the regulatory landscape of the insertion site and that gene clusters are often maintained to allow the sharing of regulatory sequences, we suggest that the Armcx gene cluster is globally regulated as Armcx gene expression is similar. Furthermore, we hypothesize that the evolution of this cluster was linked to the increase in the complexity of the Eutherian brain, thus adding further molecular complexity to the regulation of mitochondrial trafficking, specifically in the nervous system of higher vertebrates. In addition to putative mitochondrial targeting sequences, all Armcx / Arm10 genes contain nuclear localization signals and up to six Arm repeats at the C-terminal region. Several members, including Alex3, have nuclear localization in neurons. This observation is consistent with a previous study showing interaction of Alex3 with the transcription factor Sox10 and enhancement of its transcriptional activity by Alex3 [22] . These observations support that Armcx genes have biological functions in two compartments (namely, mitochondria and nucleus), as has been shown for other proteins, including Sox10, DISC1 and HDAC1 [39] , [40] , [41] . Finally, because of their transcriptional control [22] and the presence of six Arm domains, Armcx / Arm10 genes may functionally interact with the Wnt/β-catenin pathway. The observation that the lack of the N-terminal region targets Alex3 to the nucleus and the existence of a putative starting codon at the first internal methionine (aa 38) raise the possibility of alternatively translated isoforms acting selectively at the mitochondria or in the nucleus. Our data suggest that Alex3 protein is not involved in mitochondrial respiration, DNA copy number determination, mitochondrial membrane potential regulation, or Ca 2+ homoeostasis and handling in mitochondria. This is interesting because often proteins regulating mitochondrial dynamics also participate in these bioenergetic processes [28] . Similarly, we were unable to find evidence of the involvement of Alex3 in mitochondrial fusion. Thus, our data suggest that the Armcx / Arm10 genes constitute a new family of proteins specifically engaged in mitochondrial dynamics and trafficking and in mitochondrial/nuclear communication. Alex3 causes mitochondrial aggregation and/or tethering, and this effect is independent of the levels of Miro1, a protein involved in mitochondrial aggregation [32] , [33] . These findings suggest that Alex3 regulates aggregation by an as yet unknown mechanism, which is likely to involve interaction with proteins that control tethering and aggregation, including Mitofusins [28] . It has been reported that Arm motifs of p115 protein bind the Rab1 GTPase controlling ER to Golgi trafficking and regulate vesicle tethering [42] . Mitochondrial aggregating phenotypes have been observed after dysfunction of Miro and Trak2 proteins, suggesting that alteration of transport results in aggregation [43] , [44] . In neurons, mitochondrial aggregation and tethering is believed to serve to capture these organelles at specific locations requiring high-energy and Ca 2+ buffering conditions [43] , [45] . At least one of the Armcx genes ( Alex3 ) interacts with the KIF5/Miro/Trak2 complex, which controls mitochondrial dynamics in neurons in a Ca 2+ -dependent manner. Our immunoprecipitation experiments show that Alex3 interacts directly with Miro1-2 and Trak2. However, we were unable to find a direct interaction with the Kinesin motor KIF5. Importantly, the interaction of Alex3 with Miro/Trak2 proteins requires low Ca 2+ concentrations, as the presence of Ca 2+ dramatically reduced the interaction. Furthermore, mutation of the EF-hand motif in Miro1 protein abolished this Ca 2+ dependence, thereby indicating that Ca 2+ -driven conformational changes in Miro proteins [10] , [11] , [46] are the essential mechanisms that regulate the interaction between Alex3 and the Miro/Trak2 complex. Thus, while low Ca 2+ concentrations may favour the formation of KIF5/Miro/Trak2/Alex3 complexes, increases in intracellular Ca 2+ rapidly uncouple such complexes (including Alex3), thereby arresting mitochondrial trafficking. Our experiments indicate that the C-terminal region containing six Arm domains is required to interact with Miro protein. However, we do not yet know whether this interaction is mediated directly by these domains, as is the case for other proteins [47] , or by other regions included in the C-terminus. The notion that Alex3 interacts with the Miro/Trak2 complex when mitochondria are motile at low Ca 2+ concentrations [10] , [11] is further supported by our findings that knockdown of Alex3 results in a decrease in the percentages of motile mitochondria, similarly to what was observed in Miro/Trak2 loss-of-function [10] , [31] , [48] . The observation that knockdown of Alex3 does not affect the speed of the few motile mitochondria present suggests a mechanism in which Alex3 favours the formation of KIF5/Miro/Trak2 complexes (thereby enhancing mitochondrial trafficking). However, Alex3 is unlikely to be involved in regulating the motor activity of Kinesin itself. We consider our Alex3 overexpression findings, in which both the percentage and velocity of motile mitochondria were reduced, to provide further evidence of the physiological involvement of this protein in mitochondrial trafficking, possibly by deregulating and/or recruiting components of the complex (acting as a dominant negative). Together with our biochemical data, the present functional study proposes a model in which Alex3 protein is a positive regulator of mitochondrial trafficking, by interacting directly with Miro/Trak2. Furthermore, as shown for the KIF5/Miro/Trak2 complex [10] , [11] , increased neuronal activity leading to increases in Ca 2+ is likely to cause Alex3/Miro/Trak2 complex disassembly and mitochondrial arrest at active neurotransmission sites, thereby fulfilling the bioenergetic requirements of neuronal transmission. In conclusion, here we describe a new family of genes organized in a genomic cluster encoding proteins targeted to mitochondria that regulates mitochondrial dynamics and trafficking in neurons, and interacts with the KIF5/Miro/Trak2 complex. Importantly, the Armcx cluster emerged suddenly during the early evolution of Eutheria. We thus propose a further complexity in the molecular mechanisms controlling mitochondrial dynamics, specifically in the neurons of more evolved brains. Our data point to relevant functions of the Armcx gene cluster in the function of the nervous system and a novel link between mitochondrial dynamics and brain complexity. DNA analyses Armcx DNA sequences, protein translation and chromosomal linkage analyses were performed by browsing public genome data ( www.ensembl.org , www.ncbi.nlm.nih.gov ) and manual curation through analysis and BlastN of EST databases in NCBI as well as by reciprocal blasting between mammalian orthologs. Domain structure was determined by NCBI, Prosite, InterProScan, IPSort, HHPred and Wolfsort software. Phylogenetic trees were made by Bayesian methods using MrBayes 3.1.2 [49] . Plasmid vectors Alex3 full sequence was obtained by screening a P0 mouse brain cDNA library (Stratagene). For the generation of Alex3, Alex3–myc and GFP–Alex3Δ(1–12) expression vectors, pBluescript–Alex3 was subcloned into the desired expression vectors: pcDNA.3 (Invitrogen, Carlsbad, CA, USA), pSecTag-A (Invitrogen), and pEGFP-N3 and pEGFP-C1 (Clontech). For the generation of Alex3–GFP, Alex3(1–200)–GFP, Alex3(1–106)–GFP and Alex3(1–45)–GFP , Alex3 was amplified with high-fidelity Pfu, and a BamHI restriction site was introduced by using appropriate primers (Forward: 5′-CTATAGGGCGAATTGGGTACCG-3′; and reverse: for Alex3–GFP 5′-GGATCCTTCCTGACTCTTTGGGAACATCC-3′; for Alex3(1–200)–GFP 5′-GGATCCAAGCCTGCGCTGATTTTCGG-3′ and for Alex3(1–45)–GFP 5′-GGATCCATCACCAGAGCCACCCTCA-3′). All the constructs were sequenced with BigDye-Terminator v3.1 (Applied Biosystems). shRNAi sequences were designed against the Alex3 messenger RNA sequence using siRNA primer designer software v1.51 (Promega) and subcloned into pLVTHM vector (Tronolab) through MluI/ClaI (New England Biolabs) digestion. The sequence of the selected shRNAi–Alex3 was 5′-CGCGTCCCCGGCTTTAATTGTCCTAAATTTCAAGAGAATTTAGGACAATTAAAGCCTTTTTGGAAAT-3′; and the scrambled shRNAi–control 5′-CGCGTCCCCGCAGCTTTAATTGCTCTGGGTAATAATATTCATATTACCCAGAGCAATTAAAGCTGCTTTTTGGAAAT-3′. The expression vectors Miro1–myc, Miro2–myc, Miro1ΔEF–myc, KIF1C–myc and Trak2–myc were as previously described [10] , [38] . Miro1 shRNAi (V2MM_72258, TGCTGTTGACAGTGAGCGCCCTGATTGCACTACTGAATTATAGTGAAGCCACAGATGTA TAATTCAGTAGTGCAATCAGGATGCCTACTGCCTCGGA; and a control scrambled sequence) was provided by Josef Kittler (UCL, London). The mitochondrial-targeted aequorin and mito-PAGFP were as previously described [27] , [29] . MitDsRed was a gift from Antonio Zorzano (IRB Barcelona). GST–Miro1 and GST–Miro1ΔEF were kindly provided by Josef Kittler [10] . Animals All procedures were performed in accordance with the guidelines approved by the Spanish Ministry of Science and Technology and following the European Community Council Directive 86/609 EEC. OF1 embryos and postnatal mice (Iffra Credo, Lyon, France) were used. The mating day was considered embryonic day 0 (E0) and the day of birth postnatal day 0 (P0). The following developmental stages were studied: E9, E10, E11, E12, E16, P6 P21 and adult. Animals were anesthetized with 4% halothane before killing. Histological and in situ hybridization techniques are detailed in Supplementary Methods . Alex3 antibodies Polyclonal antibodies against Alex3 were generated by injecting rabbits with a synthesized peptide (369-LTERMFPKSQE-379). Cell culture and bioenergetic parameters HEK293AD cells were used for all the experiments. Cells were cultured in DMEM medium supplemented with 10% fetal bovine serum, 2 mM glutamine, 120 μg ml −1 Penicillin and 200 μg ml −1 Streptomycin. Upon confluence, cells were trypsinized (0.25% w/v) and plated at the desired density. After 2 days, cells were transfected using Fugene6 (Roche Diagnostics), following the manufacturer's instructions, and using a 1:1 DNA ratio when two constructs were transfected. For immunoprecipitation assays, an empty vector was used to balance transfected DNA when required. E16 mouse brains were dissected in PBS containing 0.6% glucose and the hippocampi were dissected out. After trypsin (Invitrogen) and DNAse treatment (Roche Diagnostics), tissue pieces were dissociated, and cells were seeded onto 0.5 mg ml −1 poly-l-lysine (Sigma-Aldrich)-coated coverslips (for immunocytochemistry) or 35-mm Fluorodish plates (World Precision Instruments, Inc) for live imaging in neurobasal medium (Gibco) containing 2 mM glutamax, 120 μg ml −1 Penicillin, 200 μg ml −1 Streptomycin and B27 supplement (Invitrogen), and were maintained at 37 °C in the presence of 5% CO 2 . Cells were cultured for between 7 and 15 days. Neuron transfection was carried out at 10–12 DIV for immunocytochemistry experiments and at 4 DIV for live imaging, using Lipofectamine 2000 (Invitrogen), following the manufacturer's instructions, and using a 1:3 DNA ratio when transfection of two constructs was required. Cells were processed 24–48 h after transfection. Neurite extension and branching was analysed as described [50] in three experimental groups (control–GFP, Alex3–GFP/m-Cherry and shRNAi–Alex3) Immunocytochemical and electron microscopy techniques as well as methods used to determine bioenergetic parameters and Ca 2+ handling are detailed in Supplementary Methods . Imaging and quantification of axonal transport of mitochondria HEK293AD cells and hippocampal neurons were seeded onto Poly-l-lysine-coated Fluorodish plates (World Precision Instruments, Inc), transfected with Alex3–GFP, MitDsRed or mito-PAGFP and filmed 24 to 48 h after using a Leica TCS SP2 confocal microscope (Leica Microsystems) equipped with a ×63 immersion oil objective. Methods used to determine mitochondrial fusion are detailed in Supplementary Methods . For mitochondrial aggregation in transfected HEK293AD cells, time lapse series of image stacks composed of 10 images (512×512 px) were taken every 5 min over 6 h using Leica Confocal Software (Leica Microsystems). Movies were generated at 10 frames per second. For mitochondrial fusion analyses in HEK293T cells, time lapse series of image stacks composed of seven images (512×512 px) were taken every 6 s over 15 min. Movies were generated at 7 frames per second. Axonal mitochondria were registered with an additional digital zoom of ×1.7. Time lapse series of image stacks composed of 5 images (512×512 px) were taken every 6 s during 15 min. All 151 stacks obtained were processed mainly with Leica Confocal Software. Further image processing, analysis and video compilation (10 frames per second) and edition was done with ImageJ software (version 1.43K, NIH, USA). Kymographs were generated with MetaMorph Software (Molecular Devices–MDS Analytical Technologies). In overexpression experiments, 42 axons were registered and analysed in each condition while in silencing experiments 22 axons per group were recorded. In all cases, a mitochondrion was considered motile when it moved more than 0.5 μm during 1 min of recording. Distances and speeds of retrograde and anterograde transport were measured separately from the corresponding kymographs, as previously described [51] , and no tracking–plugging was used. ImageJ software was used to quantify mitochondrial length. The first frame recorded of each video was digitally processed and thresholded (using Yi algorithm), and the longest distance between any two points along the selection boundary (Feret's parameter) was measured for all mitochondria. To ensure equal relevance between axons, independently of the number of mitochondria displayed, an average length was calculated for each neuron and then the mean was calculated between axons. Protein studies HEK293AD cells were obtained and lysed in Laemmli Buffer at 98 °C for 5 min. Brain extracts were obtained by homogenization in lysis buffer (50 mM HEPES; 150 mM NaCl; 1.5 mM MgCl 2 ; 1 mM EGTA; 10% glycerol; 1% Triton X-100; protease inhibitor cocktail (Roche Diagnostics Gmbh), 1 mM NaF, 0.5 M sodium pyrophosphate and 200 mM orthovanadate). About 20 μg of protein for each sample was loaded and run in polyacrylamide gels at 100 V. Transfer to nitrocellulose membranes was performed in 120 mM glycine, 125 mM Tris, 0.1% SDS and 20% methanol at 35V over night. Membranes were then blocked in 5% powder milk in TBS and incubated with primary antibodies anti-Alex3 (1:2000), anti-GFP (1:1000, Invitrogen), anti-myc (1:2000, Santa Cruz Biotechnologies) or anti-KHC (1:1000, Millipore). Anti-actin was used as a loading control (1:1000, Chemicon, Temecula, CA, USA). Secondary antibodies coupled to horseradish peroxidase were used diluted 1:2500 in TBS containing 5% powder milk. Labelling was visualized with ECL plus (Amersham Pharmacia Biotech). HEK293AD cells were lysed using a buffer containing 50 mM Tris–HCl pH7.5; 150 mM NaCl; 1.5mM MgCl 2 ; 5 mM EDTA; 1% Triton-100; 10% glycerol; protease inhibitor cocktail (Roche Diagnostics Gmbh); 1 mM NaF; 0.5 M sodium pyrophosphate and 200 mM orthovanadate. About 500 μg of total protein per sample was used for the immunoprecipitation assays. Homogenates were incubated with anti-GFP (1:500, Invitrogen) and anti-myc (1:500, Santa Cruz Biotechnology), at 4 °C o.n. overnight. All the assays were performed using protein G-Sepharose beads (Sigma-Aldrich) for 2 h at 4 °C. The assays performed in the presence of Ca 2+ , EDTA and EGTA were omitted from the lysis buffer and Ca 2+ was added to a final concentration of 2 mM. After incubation with protein G-Sepharose, samples were washed five times in washing buffer (10 mM Tris–HCl pH8, 500 mM NaCl, 1 mM EDTA, 1 mM EGTA, 1% Triton X-100 and 0.5% NP-40) in which EDTA and EGTA were again substituted by 2 mM Ca 2+ when required. Laemmli Buffer was added to the beads and they were then boiled at 98 °C for 5 min. Proteins were then analysed by SDS–PAGE and WB. Miro1-binding assay GST fusion proteins (GST–Miro1 and GST–Miro1Δ EF) were produced in E. coli and purified as described [52] . Brain lysates (adult brain) were solubilized in a buffer containing 50 mM HEPES, 125 mM NaCl, 1% Triton, 2 mM EDTA, 3 mM EGTA, 1 mM PMSF and antipain, pepstatin and leupeptin at 10 mg ml −1 . GST fusion proteins coupled to Sepharose beads (30 μg) was exposed to 20 mg of brain lysate with varying concentrations of [Ca 2+ ]. Bound material was washed five times in the above buffer before elution with SDS sample buffer. WB was carried as described above. Statistical analysis Data were analysed with the Igor Pro (WaveMetrics) and Origin 5.0. (Microcal Software) using the Student's t test or the Mann–Whitney–Wilcoxon test for non-parametric data. Statistical significance was fixed at P <0.05; * indicates P <0.05, ** P <0.01 and *** P <0.001. How to cite this article: López-Doménech, G. et al . The Eutherian Armcx genes regulate mitochondrial trafficking in neurons and interact with Miro and Trak2. Nat. Commun. 3:814 doi: 10.1038/ncomms1829 (2012).